Mediatorless high-power glucose biofuel cells based on compressed carbon nanotube-enzyme electrodes Enzymatic fuel cells use enzymes to produce energy from bioavailable substrates. However, such biofuel cells are limited by the difficult electrical wiring of enzymes to the electrode. Here we show the efficient wiring of enzymes in a conductive pure carbon nanotube matrix for the fabrication of a glucose biofuel cell (GBFC). Glucose oxidase and laccase were respectively incorporated in carbon nanotube disks by mechanical compression. The characterization of each bioelectrode shows an open circuit potential corresponding to the redox potential of the respective enzymes, and high current densities for glucose oxidation and oxygen reduction. The mediatorless GBFC delivers a high power density up to 1.3 mW cm −2 and an open circuit voltage of 0.95 V. Moreover, the GBFC remains stable for 1 month and delivers 1 mW cm −2 power density under physiological conditions (5×10 −3 mol l −1 glucose, pH 7). To date, these values are the best performances obtained for a GBFC. The emergence of biofuel cells is driven by the need for clean methods of producing electricity from renewable fuel sources, and the ever-increasing depletion of fossil fuels. The design of biofuel cells involves the application of enzymes or microorganisms as catalyst for the targeted oxidation and reduction of specific fuel and oxidizer substrates at both electrodes to generate an electrical power output. In contrast to fuel cells, noble materials (platinum, nickel...) used in the conventional fuel cells are thus not necessary and are replaced by biological catalysts. Electricity is mainly generated from the oxidation of biofuels, such as glucose, glycerol or ethanol, coupled to the reduction of dioxygen to water. The advantage of biofuel cells lies in the aspects of enzymatic catalysis, namely activity at near-room temperature and neutral pH and selectivity [1] . Biofuels such as glucose can be found in vegetable and animal fluids, thus opening up opportunities for energy production from plants [2] and physiological fluids after the implantation of biofuel cells in the human body [3] . However, in contrast to fuel cells, Glucose Biofuel Cells (GBFCs) suffer from severe limitations such as low power output and instability over time. In addition, most of the performances of GBFCs are reported at substrate saturating conditions. Furthermore, the dioxygen and glucose concentrations in physiological fluids are markedly lower than those corresponding to the saturating glucose oxidase (GOx) conditions or the dioxygen solubility in water. As these substrate concentrations in vivo are within the concentration range where the rate of enzyme catalysis is linearly proportional to the substrate concentration, the latter constitutes a key factor limiting the GBFC power. The design of more powerful GBFCs is thus one of the major challenges for supplying implanted biomedical devices such as micropumps or artificial organs. A GBFC consists of two bioelectrodes modified with immobilized enzymes catalysing the oxidation of glucose at the anode, mainly by GOx, and the reduction of dioxygen at the cathode via laccase or bilirubin oxidase. The concomitant oxidation and reduction processes at the electrodes yield electrical power. To date, the aim in biofuel cell research has been the achievement of direct electron transfer (DET) between the redox active sites of enzymes and the electrode [4] , [5] . The majority of enzymatic fuel cells in the literature employ redox-active species with low molecular weight as mediators to establish an electron transfer between enzymes and electrodes [6] , [7] , [8] . Mediators like osmium complexes [9] , [10] , [11] , 2,2′-azino-bis(3-ethylbenzthiazoline)-6-sulfonic acid [6] and ferrocyanide allow the fabrication of a GBFC that is able to deliver some hundreds of microwatts per cm (refs 2 , 12 , 13 ). However, the immobilization of a mediator often involves complicated procedures and a decrease of the theoretical open-circuit potential (OCP) of the GBFC based on the potential difference between the prosthetic sites of the two types of enzymes involved. Furthermore, its use implies important technical issues: the mediator instability can affect directly GBFC performances over time [14] ; its leakage from the electrode may provoke toxic issues, especially in the case of implanted GBFCs; and the need for synthetic steps is a major issue for industrial applications and overall cost of the biofuel cell. Hence, considerable attention has recently been given to enzymatic biofuel cells based on DET [15] , [16] , [17] , [18] . By using DET between an enzyme and an electrode, biofuel cells can operate close to the thermodynamic redox potential of the enzyme and, thereby, maximizing the OCP. Carbon nanotubes (CNTs) have diameters in the range of a few nanometers, high chemical and electrochemical stability and excellent electrical conductivity. For these reasons, CNTs are considered as ideal conducting nanowires to establish efficient DET between the active site of an enzyme and the electrode surface. CNTs were thus added to different kinds of composite electrode materials to improve the matrix conductivity or even to display DET [19] . However, for GBFCs based on CNTs, the best performances for DET led to unexpected weak power values (1 to 10 μW cm −2 in human serum) [20] , [21] whereas the best performance for mediated electron transfer, reported by Mano and co-workers, reached 740 μW cm −2 in the presence of 0.015 mol l −1 glucose [10] . We have recently shown the implantation of a GBFC in rats [3] . These graphite-based electrodes were stable for 40 days in the extracellular fluid but only delivered 5 μW cm −2 , a value that is still far from that which is required to supply implanted devices. With the aim of enhancing the GBFC power yield, we report here a convenient and straightforward approach of bioelectrode fabrication using CNTs that allows a direct electrical wiring of GOx and laccase. Thus, three-dimensional CNT bioanodes and biocathodes were fabricated by mechanical compression of CNTs and enzymes. In contrast to the functionalization of electrode surfaces by CNT deposits, this method consists of creating bioelectrodes directly from the CNT and enzymes. In addition, the entrapment of enzymes within the CNT matrix ensures an efficient electrical wiring of the redox sites of the enzyme by the surrounding CNTs. The performance of the resulting GFBCs is superior to those previously reported in the literature. Bioelectrode fabrication Bioanodes and biocathodes were fabricated by respectively mixing laccase (12.5–90 mg) and GOx (50 mg) with multi-walled carbon nanotubes (MWCNTs) (250 mg) and water (1 ml) to obtain a homogeneous composite material. The disks were prepared by compacting the composite material under applied force of 1×10 4 N in a hydraulic press (Perkin–Elmer). The resulting disks are 3 mm thick and 13 mm in diameter. Insulating water-repellent glue was used to cover the electrode leaving one side open (surface 1.3 cm 2 ). This side was finally covered with a cellulose film to prevent any enzyme or nanotube diffusion out of the electrode into the electrolyte. 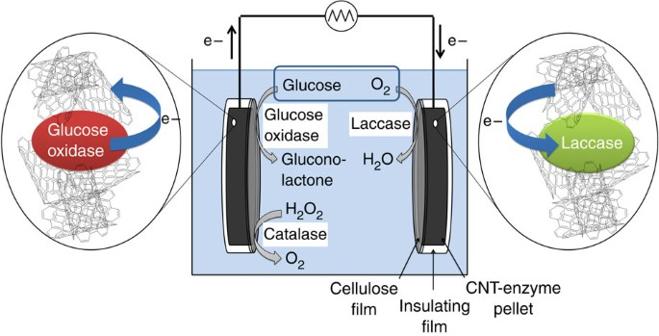Figure 1: Schematic presentation of the setup of a GBFC. At the anode, glucose is oxidized to gluconolactone, where the electrons are transferred from the GOX to CNT. Catalase decomposes hydrogen peroxide into oxygen and water. At the cathode, electrons are transferred from CNT to laccase where dioxygen is reduced to water. The biofuel cell, depicted in Figure 1 , was finally assembled by coupling one disk containing laccase to one disk containing GOx. No membrane was needed to separate anodic and cathodic compartments. Figure 1: Schematic presentation of the setup of a GBFC. At the anode, glucose is oxidized to gluconolactone, where the electrons are transferred from the GOX to CNT. Catalase decomposes hydrogen peroxide into oxygen and water. At the cathode, electrons are transferred from CNT to laccase where dioxygen is reduced to water. Full size image At the anode, it is expected that CNTs can electrically connect the entrapped GOx and thus catalyse the oxidation of glucose to gluconolactone with no need of redox mediator for the electron transfer from the redox enzyme. Due to the presence of dioxygen, a possible parasitic regeneration of non-wired GOx by O 2 can lead to the formation of hydrogen peroxide whose accumulation inside the matrix may be deleterious for GOx. To overcome the issue of peroxide contamination, catalase was added to the Gox–CNT mixture before compression to decompose H 2 O 2 . In this vein, DET was expected at the cathode between laccase and MWCNTs to achieve the bioelectrocatalytic reduction of dioxygen. The morphology of bioelectrodes was studied by Scanning Electron Microscopy (SEM). 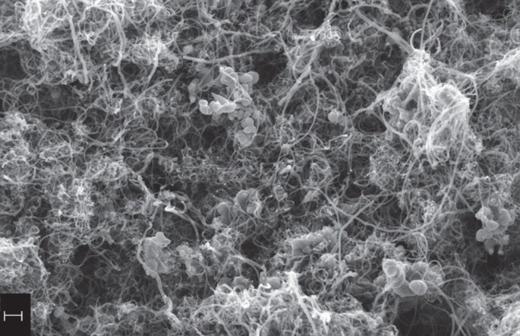Figure 2: SEM micrograph of a cross-section of the bioanode. The scale bar corresponds to 200 nm. The SEM micrograph in Figure 2 shows the cross-section of the bioanode. Even if single proteins cannot be observed, enzyme agglomerates are found distributed all over the CNTs framework, suggesting homogenously dispersed biomolecules within the CNT matrix. A specific BET surface area of 180 m 2 g −1 and a void fraction of 43% were measured for these bioelectrodes. As expected, the MWCNT electrodes exhibit a high surface area and a high porosity. Figure 2: SEM micrograph of a cross-section of the bioanode. The scale bar corresponds to 200 nm. Full size image Biocathode characterization The performances of the bioelectrodes were examined in phosphate buffer (0.1 M, pH 7, 20 °C). The OCP values vary between 0.50 and 0.58 V versus saturated calomel electrode (SCE) depending on the amount of enzyme incorporated in the CNT disk. The chronoamperometric response of the biocathode was recorded at 0 V versus SCE with and without dioxygen. The appearance of a strong cathodic current (−4.4 mA cm −2 ) that corresponds to the catalytic reduction of dioxygen by laccase confirms the presence of immobilized enzymes and retention of their activity ( Fig. 3a ). It should be noted that the same experiment carried out with a similar biocathode without laccase exhibited no current response, thus excluding the possible contribution of the nanotubes to the catalytic reduction of dioxygen. 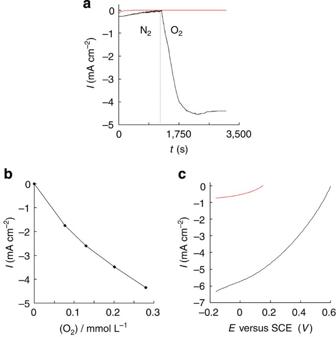Figure 3: Biocathode performances. (a) Chronoamperometric response for biocathode (red) without laccase, (black) with 20% laccase, in N2saturated solution and after saturation with dioxygen at 0 V versus SCE. (b) Amperometric response at the biocathode (20% laccase) potentiostated at 0 V as a function of dioxygen concentration. (c) Polarization curves of the biocathode, (red) without laccase and (black) with 20% laccase, in air-saturated solution (2 mV s−1scan rate). Experiments carried out in air-saturated phosphate buffer 0.1 mol l−1, pH 7.0. Figure 3b shows the biocathode response as a function of dioxygen concentration. It appears that the current density increases linearly with the dioxygen concentration corroborating the catalytic character of this current towards the dioxygen reduction. Figure 3c presents the polarization curves related to CNT electrodes with and without laccase. Between 0.58 and −0.15 V versus SCE, the catalytic reduction current (in absolute value) recorded at the biocathode increases continuously to a maximum value of −6.2 mA cm −2 . In contrast, the CNT electrode displays a reduction current only at 145 mV, which reaches −0.74 mA cm −2 at −0.15 V, highlighting the importance of the electroenzymatic reaction. Figure 3: Biocathode performances. ( a ) Chronoamperometric response for biocathode (red) without laccase, (black) with 20% laccase, in N 2 saturated solution and after saturation with dioxygen at 0 V versus SCE. ( b ) Amperometric response at the biocathode (20% laccase) potentiostated at 0 V as a function of dioxygen concentration. ( c ) Polarization curves of the biocathode, (red) without laccase and (black) with 20% laccase, in air-saturated solution (2 mV s −1 scan rate). Experiments carried out in air-saturated phosphate buffer 0.1 mol l −1 , pH 7.0. Full size image Different amounts of laccase were incorporated into the CNT disks by keeping the amount of MWCNT constant, to optimize the biocathode performances ( Fig. 4a ). At 0 V, the catalytic current density increases from −2 to −5.8 mA cm −2 with increasing amount of immobilized laccase from 2 to 20% reaching a constant value (−5.8 mA cm −2 ) for higher laccase loading. Similarly, the OCP increases from 0.50 to 0.58 V with increase in laccase loading and becomes stable above 20% wt laccase. This OCP increase might be ascribed to the effect of the hydrophobic character of the CNT matrix on the redox potential of laccase [22] , [23] . The potential change may result from a decreasing hydrophobic microenvironment of the compressed enzyme induced by the increasing percentage of enzymes in the CNT disk. Moreover, this changing hydrophobicity/hydrophilicity ratio of the CNT disk may also alter the diffusion of aqueous buffer to the trapped enzyme and thus lead to different local pH values during the enzymatic conversion of oxygen [24] . The measured OCP (0.58 V) corresponds to the laccase redox potential [25] and underlines the electrical wiring of laccase without any overpotential. Such high current densities and the absence of overpotential indicate the excellent electrical wiring of the immobilized enzyme to the electrode. Moreover, the mechanical stability of the biocathode, and hence the reproducibility and stability of electrical wiring system was evaluated by periodically measuring OCP and current density at 0 V for 30 days ( Fig. 4b ). After an initial decrease during the first 3 days, both OCP and current density remained stable with respective values of 0.55 V and 3.8 mA cm −2 . With the aim to develop implantable GBFC and hence to operate in physiological conditions, we performed all experiments at pH 7. It is noteworthy that, although the optimum pH of laccase is pH 4, we did not observe any decrease in performance at pH 7 over 30 days. We also studied the possible inhibition of laccase by chloride ions. For this purpose, the amperometric response of the biocathode was investigated at different NaCl concentrations close to physiological conditions. We observed a low decrease of the current density above 50 mM NaCl. At 150 mM NaCl (concentration in human serum), the current density decreased by only 5% compared with the initial value of the catalytic current ( Supplementary Figure S1 ). This indicates the high stability of wired laccase towards chloride inhibition. 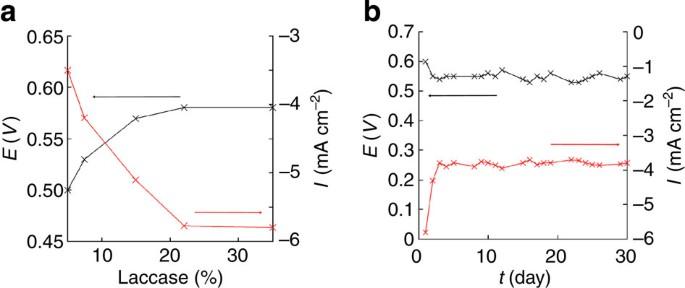Figure 4: Influence of the laccase loading and operational time on the biocathode performance. (a) Evolution of OCP (black) and current density (red) at 0 V, with different amounts of laccase (mass percentage in the electrode) in air-saturated solution. (b)Evolution of OCP (black) and current density (red) at 0 V, of biocathode (20% laccase) versus time. Experiments carried out in air-saturated phosphate buffer 0.1 mol l−1, pH 7.0. Figure 4: Influence of the laccase loading and operational time on the biocathode performance. ( a ) Evolution of OCP (black) and current density (red) at 0 V, with different amounts of laccase (mass percentage in the electrode) in air-saturated solution. ( b )Evolution of OCP (black) and current density (red) at 0 V, of biocathode (20% laccase) versus time. Experiments carried out in air-saturated phosphate buffer 0.1 mol l −1 , pH 7.0. Full size image Bioanode characterization To overcome the parasitic regeneration of GOx by dioxygen and concomitant H 2 O 2 production, we incorporated catalase into the bioanode; this enzyme catalyses H 2 O 2 disproportionation into O 2 and water. The enzymatic removal of H 2 O 2 prevents its electrochemical reduction at the nanotube disk that would create at the bioanode a mixed potential between those of glucose oxidation event and H 2 O 2 reduction. Effectively, it appears that the OCP of the GOx bioelectrode was affected by the amount of co-immobilized catalase. Its value shifted to negative values from −0.20 to −0.43 V with increasing catalase loading. The bioanode, potentiostated at −0.1 V, exhibits an anodic current response to successive glucose additions (5 mmol l −1 ) indicating the retention of GOx activity in the compacted CNT matrix ( Fig. 5a ). As expected, no amperometric response was recorded in absence of GOx in the pressed CNT disk. 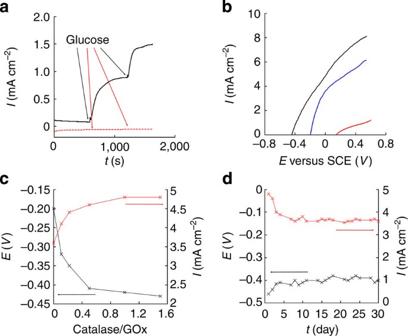Figure 5: Bioanode performances. (a) Chronoamperometric response for bioanode (red) without enzymes and (black) with GOx and catalase (catalase/GOx ratio 1:1); after two successive additions of 0.005 mol l−1glucose, at −0.1 V. (b) Polarization curves of bioanode (red) without enzyme, (blue) with GOx (black) with GOx and catalase (catalase/GOx ratio 1:1); in 0.05 mol l−1glucose solution (2 mV s−1scan rate). (c) Evolution of OCP (black) and current density (red) at 0 V, versus catalase/GOx ratio in bioanode, in 0.05 mol l−1glucose solution. (d) Evolution of OCP (black) and current density (red) of bioanode (catalase/GOx ratio 1:1) at 0 V versus time, in 0.05 mol l−1glucose solution. Experiments carried out in air-saturated phosphate buffer 0.1 mol l−1, pH 7.0. Figure 5: Bioanode performances. ( a ) Chronoamperometric response for bioanode (red) without enzymes and (black) with GOx and catalase (catalase/GOx ratio 1:1); after two successive additions of 0.005 mol l −1 glucose, at −0.1 V. ( b ) Polarization curves of bioanode (red) without enzyme, (blue) with GOx (black) with GOx and catalase (catalase/GOx ratio 1:1); in 0.05 mol l −1 glucose solution (2 mV s −1 scan rate). ( c ) Evolution of OCP (black) and current density (red) at 0 V, versus catalase/GOx ratio in bioanode, in 0.05 mol l −1 glucose solution. ( d ) Evolution of OCP (black) and current density (red) of bioanode (catalase/GOx ratio 1:1) at 0 V versus time, in 0.05 mol l −1 glucose solution. Experiments carried out in air-saturated phosphate buffer 0.1 mol l −1 , pH 7.0. Full size image Figure 5b shows the polarization curves recorded using a (black) catalase/GOx MWCNT bioelectrode, (blue) a GOx MWCNT bioelectrode, and (red) an enzyme free MWCNT electrode. All these bioanodes were soaked in phosphate buffer (pH 7.0) containing glucose (0.05 mol l −1 ). For the catalase/GOx bioanode, the anodic current increases with increasing potential between −0.41 V and +0.58 V, reaching a high current density close to 8 mA cm −2 . This value confirms the high electrocatalytic activity of the wired GOx and the negligible GOx regeneration by dioxygen. Polarization curves recorded for the bioanode, with and without catalase, confirmed the important role of catalase in decreasing the OCP and increasing current density of the bioanode ( Fig. 5b ). Indeed, in the presence of catalase, the OCP decreases from −0.20 V to −0.43 V. Without catalase, the presence of H 2 O 2 involves a mixed potential at the anode and, consequently, a decrease of anodic current (about 20%) is observed. Furthermore, as observed for the biocathode, no catalytic current was detected for the enzyme-free MWCNT electrode between −0.43 and +0.14 V, demonstrating the lack of reactivity of MWCNT for the glucose oxidation. The catalase/GOx ratio was optimized to ensure optimal H 2 O 2 disproportionation. Figure 5c shows the evolution of OCP and the catalytic current density (at 0 V) as a function of catalase/GOx ratio. As mentioned above, the OCP decreases with increasing catalase/GOx ratio from −0.20 to −0.43 V. Above the ratio 1/1, the OCP (−0.43 V) corresponds to the redox potential of GOx [26] , indicating that H 2 O 2 was rapidly decomposed and does not affect the oxidation potential. Furthermore, the current density increases from 3.6 mA cm −2 up to 4.8 mA cm −2 with increasing catalase/GOx ratio. This high anodic current response to glucose, combined with an OCP close to the redox potential of the flavin adenine dinucleotide entrapped within Gox, indicates an efficient DET between GOx and the surrounding MWCNT matrix. Moreover, the evolution of the anodic current response and OCP of the bioanodes as a function of time also exhibits a 25% decrease of the initial current intensity and a positive shift of only 60 mV for the OCP after 30 days. This illustrates the good stability of the biocomposite disk ( Fig. 5d ). Glucose BioFuel cell characterization A glucose/dioxygen biofuel cell was then elaborated by associating bioanode and biocathode without a separating membrane. 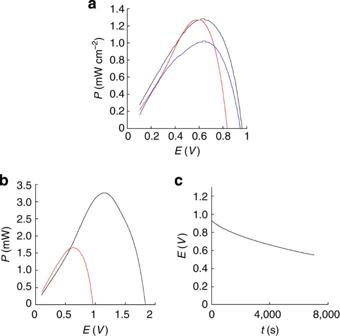Figure 6: GBFC performances. (a) Dependence of power density on operating voltage in 0.05 mol l−1glucose solution before (black) and after one month (red). Blue curve: dependence of power density on operating voltage in 5 × 10−3mol l−1glucose. (b) Dependence of power on operating voltage in 0.05 mol l−1glucose solution for one GBFC (red) and two GBFCs connected in series (black). (c) Dependence of voltage on time for continuous discharge under 200 μA cm−2in 0.05 mol l−1glucose solution. Experiments carried out in air-saturated phosphate buffer 0.1 mol l−1, pH 7.0 (bioanode: catalase/GOx ratio 1:1, biocathode: 20% laccase). Figure 6a shows the performances of the resulting GBFC, operating at room temperature (20 °C) in phosphate buffer (pH 7) containing 0.05 mol l −1 glucose. As expected, the recorded OCV of 0.95±0.05 V corresponds to the difference between the individually measured OCPs of the biocathode and the bioanode. This value represents, to the best of our knowledge, the highest OCV reported for a GBFC. The variation of the power density as a function of the cell voltage presents the typical bell-shaped curve relative to a fuel cell with a maximum of 1.3 mW cm −2 at 0.6 V. This power density dependence on the cell voltage was recorded after 30 days storage of GBFC in the buffer solution leading to a 4% decrease for the maximum power density that reaches 1.25 mW cm −2 at 0.57 V ( Fig. 6a , red curve). As observed for both, the biocathode and bioanode separately, an OCP decrease of 0.1 V is observed in the first hours of the experiments. This probably arises from an equilibration step that involves the diffusion of the electrolyte inside the porous electrodes and the pH stabilization at the enzyme/electrode interface. After one day, both power density and OCP remain stable for 30 days, the biofuel being kept in the buffer solution at room temperature. Figure 6a (blue curve) shows the performances of the GBFC in phosphate buffer containing 5×10 −3 mol l −1 glucose that corresponds to the concentration of glucose in extracellular body fluids. Even at low glucose concentration, the GBFC exhibits excellent performances (OCV=0.93±0.05 V and maximum power density=1.0 mW cm −2 ). Figure 6: GBFC performances. ( a ) Dependence of power density on operating voltage in 0.05 mol l −1 glucose solution before (black) and after one month (red). Blue curve: dependence of power density on operating voltage in 5 × 10 −3 mol l −1 glucose. ( b ) Dependence of power on operating voltage in 0.05 mol l −1 glucose solution for one GBFC (red) and two GBFCs connected in series (black). ( c ) Dependence of voltage on time for continuous discharge under 200 μA cm −2 in 0.05 mol l −1 glucose solution. Experiments carried out in air-saturated phosphate buffer 0.1 mol l −1 , pH 7.0 (bioanode: catalase/GOx ratio 1:1, biocathode: 20% laccase). Full size image To underline the possible use of our GBFC to supply electronic devices and, in particular, implanted biomedical devices that usually require at least an operating voltage of 0.5–0.6 V, we connected two GBFC in series ( Fig. 6b , black curve) and obtained an OCV of 1.8 V with a maximum power of 3.25 mW at 1.2 V. This clearly shows that our strategy of bioelectrode construction can be used to develop GBFCs that are able to supply electronic devices that work at voltage up to 1.2 V by connecting two GBFCs in series. Finally, we studied the evolution of the GBFC voltage under a constant current discharge of 200 μA cm −2 ( Fig. 6c ). Although the voltage decreased slowly to 0.6 V after two hours, these biofuel cells were able to maintain the current discharge. The high performance of our developed GBFC relies on the bioelectrode configuration that allows enzymes to operate in a three-dimensional conductive environment, as depicted in Figure 1 . The measurements of the specific BET surface area and the void fraction gave values in the order 180 m 2 g −1 and 43%, respectively. This confirms the high porosity of the electrodes and is in good agreement with the theoretical external specific surface area of MWCNT within the range 70–300 m 2 g −1 (ref. 27 ). Chronoamperometric measurements were performed with [Ru(NH 3 ) 6 ]Cl 3 as redox probe, to estimate the electroactive area of the disks. The MWCNT electrodes exhibit approximately an electroactive area of 52 cm 2 for an interfacial geometrical area of 1.3 cm 2 and a volume of 0.39 ml, providing an electrochemical specific surface area of 160 cm 2 g −1 . Taking into account that the measured specific surface area of MWCNT is 180 m 2 g −1 , these enzyme-CNT disks exhibit an electroactive area corresponding to approximately 0.01% of the experimentally determined BET surface area. Moreover, these porous bioelectrodes are highly conductive with a homogeneous conductivity of 3300 S m −1 , measured by a four-point technique. Thus, MWCNT electrodes constitute a porous matrix with a high electrical conductivity that may ensure a good diffusion for the enzyme substrate and the electrical connection of a large amount of entrapped enzymes. Moreover, the compression of the enzyme nanotube mixture likely favours a close proximity at the nanoscale level between nanotube and prosthetic sites of enzymes, leading thus to DET without any loss of activity. It is noteworthy that these physical constraints over the enzymes might also provoke partial unfolding of proteins during the fabrication process while maintaining their activity. The apparent enzyme activity was estimated from the current density values recorded for both bioelectrodes. The apparent specific activity of the wired-enzymes was compared with the activity of free enzymes in solution ( Supplementary Figure S2 ). It appears thus that the biocathode exhibits a surface activity of 3.84 U cm −2 that corresponds to a specific activity of 0.1 U mg −1 for the electrically connected laccase. Taking into account that the specific activity of laccase at pH 7 is 1 U mg −1 , the immobilized electro-enzymatic activity corresponds to 10% of the activity displayed by an equivalent amount of free enzymes in solution. The bioanode presents an electro-enzymatic activity of 2.48 U cm −2 corresponding to a specific GOx activity of 65 mU mg −1 . This activity represents 0.065% of that determined using the same amount of GOx in solution. These results are in good agreement with the decrease of enzymatic activity observed during the production of enzymatic biosensors. This loss of activity is attributed to the immobilization of enzymes. Compared with similar configurations [20] , [21] , these performances represent an increase of two to three orders of magnitude in terms of power density. Moreover, this GBFC exhibits long-term stability for a biofuel cell, maintaining a significant power output during 30 days storage. As volume and weight of a biofuel cell are also important parameters for evaluating its potentialities, the performance of the biofuel cell described here (maximum power output of 1.25 mW cm −2 ) was expressed in volumetric power and specific power, namely 1.66 mW ml −1 and 1.85 mW g −1 . Compared with the results mentioned in the literature, our bioelectrodes supply a high catalytic current density at 5 mM glucose and 150 mM NaCl, which means that efficient DET is obtained between the entrapped enzymes and the MWCNT matrix. This leads to sufficient high voltages envisioning electrical supply of implantable electronic device in a human body where the concentration of glucose is 5×10 −3 mol l −1 . To conclude, this technique can be extended to other types of enzymes, even when the active site is located deeply inside the protein as it is the case for GOx. This straightforward bioelectrode fabrication process could lead to other biofuel cell configurations, envisioning many future applications. Chemicals Multi-walled Carbon Nanotubes (diameter 10–15 nm, length 0.1–10 μm), Glucose oxidase (GOx) from Aspergillus niger (100 U mg −1 solid), laccase from Trametes versicolor (20 U mg −1 solid) and α- D -Glucose were purchased from Sigma-Aldrich and used without further purification. α- D -Glucose was prepared in phosphate buffer 0.1 M (pH 7.0) at least 24 h before its use. Cellulose membranes were purchased from Spectrumlabs: Spectra/Por Dialysis membrane, MWCO 6–8,000 g mol −1 , flat width 32 mm, diameter 20.4 mm, vol/length 3.3 ml/cm. Instrumentation The electrochemical characterization and the biofuel cell tests were performed with an Autolab potentiostat 100 (Eco Chemie). All electrochemical experiments were carried out in a conventional three-electrode cell except for the biofuel cell experiments. A Pt wire, placed in a separate compartment containing the supporting electrolyte and a SCE were used as counter electrode and reference electrode, respectively. The morphology of bioelectrodes was characterized by SEM using an ULTRA 55 FESEM based on the GEMENI FESEM column with beam booster (Nanotechnology Systems Division, Carl Zeiss NTS GmbH) and tungsten gun. N 2 adsorption–desorption isotherms (Micromeritics -ASAP 2000) were used for analyzing the sample microstructure. The specific surface area and pore size distribution were determined by applying the BET and BJH methods respectively, to the adsorption–desorption curves. The desorption branch was used for BJH calculations. The electrical resistivity of the electrodes was measured using four-point probe configuration at room temperature on a Lucas Lab, Pro 4 instrument. How to cite this article: Zebda, A. et al . Mediatorless high-power glucose biofuel cells based on compressed carbon nanotube-enzyme electrodes. Nat. Commun. 2:370 doi: 10.1038/ncomms1365 (2011).